Elevated oncofoetal miR-17-5p expression regulates colorectal cancer progression by repressing its target geneP130 MicroRNAs (miRNAs) are essential for regulating normal embryonic development and carcinogenesis. Here we report that miR-17-5p, an oncofoetal miRNA, is a key regulator of colorectal cancer progression. We show that miR-17-5p is an oncogenic miRNA that regulates tumorigenesis and progression by targeting the gene encoding P130 and subsequently activating the Wnt/β-catenin pathway. Using specimens from two large cohorts of colorectal cancer patients, we found that patients whose tumours had high miR-17-5p expression had shorter overall survival rates but showed a better response to adjuvant chemotherapy than did patients whose tumours had low miRNA expression. We also observed a strong inverse correlation between miR-17-5p and P130 expression. The current findings suggest that miR-17-5p is a crucial determinant of colorectal cancer progression. Colorectal cancer (CRC) is the second most common cause of cancer-related mortality in the western world. There are ~600,000 new cases annually in western countries [1] . Recent decades have witnessed a rapid increase in CRC morbidity in rapidly developing countries such as China [2] . MicroRNAs (miRNAs), small non-coding RNAs that regulate the translation of many genes, are excellent biomarkers for cancer diagnosis and prognosis [3] , [4] , [5] , [6] , [7] , [8] , [9] . However, it is unclear which miRNAs are potential therapeutic and prognostic biomarkers for CRC and are associated with or regulate tumour progression. As reported in our previous studies of a potential oncofoetal CRC biomarker, certain high-value biomarkers, including miRNAs, genes and cancer proteins, show embryonic characteristics [10] , [11] , [12] , [13] . Tumorigenesis and embryogenesis have been postulated to share certain common pathways [10] . The increased proliferation and lack of differentiation of cancer cells resemble the behaviour of embryonic stem cells during the physiological process of embryogenesis. In addition, miRNAs are necessary for stem cell division, cell fate determination and patterning in the early and later stages of development, when they regulate cell differentiation and maintain pluripotency [14] , [15] , [16] . Therefore, such information may lead to the identification of specific markers for detecting CRC and of potential therapeutic targets that allow the inhibition of malignant transformation and progression. In the present study, differentially expressed oncofoetal miRNAs from foetal, cancerous and normal colorectal tissues were profiled to study their potential roles in tumour formation, prognosis and response to CRC chemotherapy. miR-17-5p was significantly upregulated in both the CRC and foetal colorectal tissues compared with the normal colorectal tissue and was chosen for further validation and analysis. Searching for oncofoetal miRNAs in CRC progression To locate oncofoetal miRNAs, we globally analysed the miRNA expression profiles of foetal colorectal tissues, CRC tissues and normal colorectal tissues using the μParaflo miRNA microarray assay. A total of 39 miRNAs were found to be expressed in the three groups ( Supplementary Table S1 ). Only one oncofoetal miRNA, miR-17-5p, was found to have a similar expression pattern in the CRC and foetal colorectal tissues but a significantly different pattern in the normal colorectal tissue ( Fig. 1a ). In addition, a cancer miRNA array was employed to calculate significant differences in the relative miRNA abundances among the three groups, and the expression pattern of oncofoetal miR-17-5p was validated ( Fig. 1a ). The validation experiments were performed using quantitative PCR with reverse transcription (qRT–PCR), and the miR-17-5p expression pattern was confirmed ( Fig. 1a ). 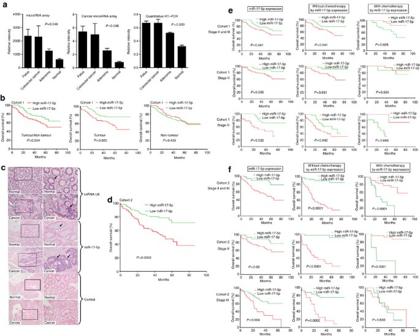Figure 1: Clinical significance of miR-17-5p expression levels in CRC patients. (a) miRNA array assays and qRT–PCR validation for miR-17-5p expression in CRC, foetal and colorectal tissues, and in tissues with varying degrees of dysplasia. (b) The miR-17-5p expression levels in cohort 1 were measured by qRT–PCR. (c) The miR-17-5p expression in colorectal epithelial cells using ISH analysis. (d) In cohort 2, high miR-17-5p expression was associated with reduced survival. (e) Associations between miR-17-5p expression and the therapeutic outcomes in stage II (n=126) and stage III (n=69) CRC patients in cohort 1 treated with adjuvant chemotherapy. (f) Associations between miR-17-5p expression and the therapeutic outcomes in stage II (n=99) and stage III (n=58) CRC patients in cohort 1 treated with adjuvant chemotherapy. All bars represent the mean values±s.d. of three experiments. Figure 1: Clinical significance of miR-17-5p expression levels in CRC patients. ( a ) miRNA array assays and qRT–PCR validation for miR-17-5p expression in CRC, foetal and colorectal tissues, and in tissues with varying degrees of dysplasia. ( b ) The miR-17-5p expression levels in cohort 1 were measured by qRT–PCR. ( c ) The miR-17-5p expression in colorectal epithelial cells using ISH analysis. ( d ) In cohort 2, high miR-17-5p expression was associated with reduced survival. ( e ) Associations between miR-17-5p expression and the therapeutic outcomes in stage II ( n =126) and stage III ( n =69) CRC patients in cohort 1 treated with adjuvant chemotherapy. ( f ) Associations between miR-17-5p expression and the therapeutic outcomes in stage II ( n =99) and stage III ( n =58) CRC patients in cohort 1 treated with adjuvant chemotherapy. All bars represent the mean values±s.d. of three experiments. Full size image Adenomas represent a CRC precursor stage. Using the μParaflo miRNA microarray assay and an miRNA cancer analysis array, we found a remarkable association between malignancy and miR-17-5p expression levels in the normal colorectal, adenoma and carcinoma tissues ( Fig. 1a ). A validation experiment was performed using qRT–PCR analysis. The results were consistent with the observations from the miRNA microarray analysis ( Fig. 1a ). High miR-17-5p expression and prognosis If miR-17-5p acts as an oncogenic miRNA, miR-17-5p overexpression should be a frequent event in CRC. Therefore, we used qRT–PCR to determine the miR-17-5p expression levels in tumour and non-tumour tissues obtained from 240 colorectal patients in cohort 1 ( Supplementary Table S2 ). To analyse the association between miR-17-5p expression and the clinicopathological characteristics of CRC patients, we used the median tumour:non-tumour ratio (T:N) to dichotomize the CRC cases. Using a high–low cutoff, we found that high T:N miR-17-5p expression ratios were associated with a shorter survival ( Fig. 1b ). This association could be due to miR-17-5p expression levels in the tumour tissue, the surrounding non-tumorous tissue or a combination of the two. To distinguish between these possibilities, we separately analysed miR-17-5p expression in tumours and paired non-tumorous tissues. High miR-17-5p expression levels in tumours were associated with a shorter survival ( Fig. 1b ). No significant associations with miR-17-5p expression were observed in the non-tumorous tissue ( Fig. 1b ). This high–low cutoff was used throughout this study. To determine whether the prognostic value of miR-17-5p expression was independent of other risk factors associated with the clinical outcome of CRC, multivariate analyses were performed using a Cox proportional hazard model. The risk factors examined included miR-17-5p expression levels, lymph node metastasis, surgical–pathological staging and others. These factors are generally known to significantly affect the CRC outcomes. In the univariate analysis, high miR-17-5p expression in tumours, TNM staging and lymph node metastases were significantly associated with survival ( Supplementary Table S3 ). In the final multivariate Cox regression model, miR-17-5p expression levels in tumours were associated with a poor survival prognosis independent of the other clinical covariates ( Supplementary Table S3 ). miR-17-5p expression in colorectal epithelial cells Although we found that high miR-17-5p expression in tumours was associated with an adverse survival outcome, those experiments did not identify the cells within a tumour that expressed miR-17-5p. To identify these cells, we used in situ hybridization (ISH) to visualize miR-17-5p expression in tumour and corresponding non-tumour tissues. miR-17-5p was expressed at higher levels in the colorectal epithelial cells of human tumour tissue than in normal tissues ( Fig. 1c ), which is consistent with miR-17-5p overexpression having a role in tumour cells during colorectal carcinogenesis. To validate the association between miR-17-5p expression and prognosis, we detected miR-17-5p expression by ISH analysis in tumour and non-tumour tissues obtained from 185 patients in cohort 2 ( Supplementary Table S2 ). Consistent with cohort 1, high miR-17-5p expression in tumours was significantly associated with poor survival ( Fig. 1d ). In a univariate analysis, high miR-17-5p expression in tumours, TNM staging and lymph node metastasis were significantly associated with survival ( Supplementary Table S3 ). In the final multivariate Cox regression model, high miR-17-5p expression in tumours was associated with a poor survival prognosis independent of other clinical covariates ( Supplementary Table S3 ). Association of miR-17-5p with tumour stages If miR-17-5p expression is causal in CRC progression, miR-17-5p expression may be associated with more advanced stages of the disease. In the current study, the more advanced tumours expressed higher levels of miR-17-5p ( Supplementary Fig. S1a ). Lymph node metastasis is also a measure of tumour progression and impacts survival in patients with solid tumours [17] . The tumours that had metastasized to the lymph nodes expressed higher miR-17-5p levels than the tumours that had not ( Supplementary Fig. S1b ). miR-17-5p expression levels and therapeutic outcome The analysis of the response to adjuvant therapy included only TNM stage II and III patients, as TNM stage I patients have an excellent survival prognosis regardless of the therapy and treatment for stage IV patients is palliative. We analysed the associations between miR-17-5p expression and the therapeutic outcomes in stage II and stage III CRC patients in cohort 1 treated with adjuvant chemotherapy. The chemotherapy regimens (with or without leucovorin, levamisole or cisplatin) were primarily fluorouracil based. The Kaplan–Meier analyses found that high miR-17-5p expression was associated with a poor prognosis in stage II and stage III patients ( Fig. 1e ), further indicating the potential role of miR-17-5p as a prognostic biomarker. The adjuvant chemotherapy was beneficial to the patients with stage II or stage III CRC, although this benefit was only significant in the stage III patients. High miR-17-5p expression was associated with favourable therapeutic outcomes in the patients with stage II or III cancer who received adjuvant therapy and in the patients with stage III cancer alone ( Fig. 1e ). The multivariate Cox regression found that high miR-17-5p expression predicted poor outcomes and that adjuvant chemotherapy was associated with a favourable survival rate independent of other clinical covariates ( Supplementary Table S4 ). A similar result was observed in cohort 2 ( Supplementary Table S4 ; Fig. 1f ). Adjuvant chemotherapy was beneficial in both the stage II and stage III CRC patients, although this benefit was only significant for the stage II patients in cohort 2. Therefore, miR-17-5p expression emerged as an independent predictor of the response to adjuvant chemotherapy. To explore the potential mechanisms that explain this phenomenon, we performed an in vitro experiment using two CRC cell lines, LoVo and SW480. We found that miR-17-5p expression levels decreased in the cells treated with fluorouracil (5-Fu) ( Supplementary Fig. S2 ). In addition, apoptosis assays confirmed that miR-17-5p suppressed apoptosis and G1 arrest; however, cell apoptosis and G1 arrest were increased in the miR-17-5p-transfected CRC cells that were treated with 5-Fu ( Supplementary Figs S3, S4, S5 and S6 ). The role of miR-17-5p in vitro and in vivo To determine the oncogenic properties of miR-17-5p, the LoVo CRC cell line was transiently transfected with an miR-17-5p mimic, an miR-17-5p inhibitor or a control. A qRT–PCR assay showed that miR-17-5p expression was significantly greater in the miR-17-5p mimic-transfected cells and lower in the miR-17-5p inhibitor-transfected cells than in the controls ( Fig. 2a ). The MTT and clonogenic assays demonstrated that suppressing miR-17-5p with an miR-17-5p inhibitor leads to a significant decrease in LoVo cell proliferation and that simulating miR-17-5p overexpression using an miR-17-5p mimic leads to a significant increase in LoVo cell proliferation ( Fig. 2b ). Apoptosis and TUNEL assays found that miR-17-5p suppressed cell apoptosis and G1 arrest ( Fig. 2d ). In addition, transwell assays found that miR-17-5p promoted both migration and invasion in the LoVo cells ( Fig. 2f ). We also performed in vitro experiments in an independent cell line, SW480 and similar results were obtained using the SW480 cells ( Supplementary Fig. S7 ). 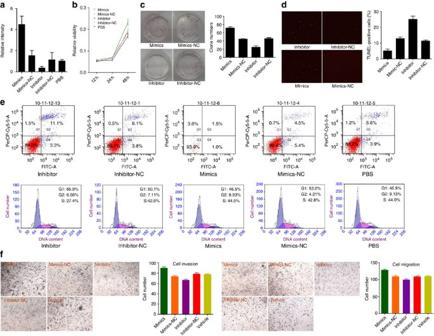Figure 2: miR-17-5p regulates proliferation and motility in LoVo cells. (a) qRT–PCR assay for miR-17-5p expression different treatment groups. (b) MTT assay for CRC cell proliferative activity in different treatment groups and different times after transfection. (c) Clonogenic assay for CRC cells proliferative activity in different treatment groups after transfection. Apoptosis (d) and TUNEL (e) assays showed that miR-17-5p suppressed cell apoptosis and G1 arrest. (f) Transwell assays found that miR-17-5p showed both of migration and invasion for LoVo cells in different treatment groups. These results are representative of at least three independent experiments. All bars represent the mean values±s.d. of three experiments. Figure 2: miR-17-5p regulates proliferation and motility in LoVo cells. ( a ) qRT–PCR assay for miR-17-5p expression different treatment groups. ( b ) MTT assay for CRC cell proliferative activity in different treatment groups and different times after transfection. ( c ) Clonogenic assay for CRC cells proliferative activity in different treatment groups after transfection. Apoptosis ( d ) and TUNEL ( e ) assays showed that miR-17-5p suppressed cell apoptosis and G1 arrest. ( f ) Transwell assays found that miR-17-5p showed both of migration and invasion for LoVo cells in different treatment groups. These results are representative of at least three independent experiments. All bars represent the mean values±s.d. of three experiments. Full size image To study the tumorigenic role of miR-17-5p in CRC, immunodeficient BALB/C mice were subcutaneously injected with SW480 cells. The mice were then treated with an intra-tumoral injection of an miR-17-5p mimic, an miR-17-5p inhibitor or a control. The tumour volumes were measured throughout the treatment course until the animals were euthanized. Suppressing miR-17-5p expression with an miR-17-5p inhibitor significantly decreased tumour growth, and overexpressing miR-17-5p with an miR-17-5p mimic significantly promote tumour growth in vivo , with no apparent toxicity at the doses used ( Fig. 3a–c ). In addition, the immunodeficient BALB/C mice were subcutaneously injected with LoVo cells to validate the current results, and similar results were obtained ( Supplementary Fig. S8 ). A proliferating-cell nuclear antigen (PCNA) immunoreactivity analysis and a TUNEL assay found that miR-17-5p promoted tumour cell proliferation and deceased apoptosis in vivo ( Fig. 3d ). Taken together, these data indicate that miR-17-5p has an important role in CRC progression. 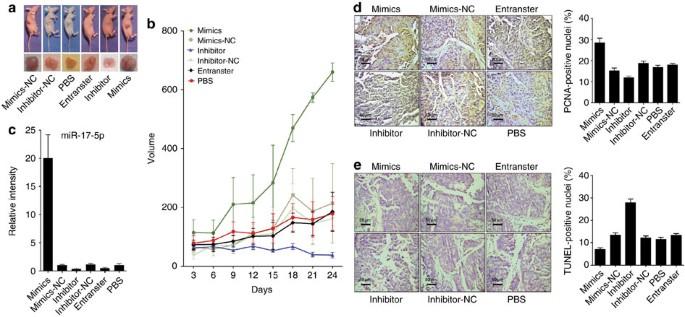Figure 3: miR-17-5p regulates tumour growth and apoptosis in CRC xenografts. (a) Images of mice bearing SW480 tumours on the 24th day after intra-tumoural injections with different treatment groups. (b) Tumour volume growth curve after intra-tumoural injections of different treatment groups over the study period. (c) qRT–PCR assay for miR-17-5p expression in different treatment groups. PCNA immunoreactivity (d) and TUNEL assay (e) for tumour cell proliferation and apoptosis in different treatment groups. These results are representative of at least three independent experiments. All bars represent the mean values±s.d. of three experiments. Figure 3: miR-17-5p regulates tumour growth and apoptosis in CRC xenografts. ( a ) Images of mice bearing SW480 tumours on the 24th day after intra-tumoural injections with different treatment groups. ( b ) Tumour volume growth curve after intra-tumoural injections of different treatment groups over the study period. ( c ) qRT–PCR assay for miR-17-5p expression in different treatment groups. PCNA immunoreactivity ( d ) and TUNEL assay ( e ) for tumour cell proliferation and apoptosis in different treatment groups. These results are representative of at least three independent experiments. All bars represent the mean values±s.d. of three experiments. Full size image miR-17-5p can downregulate P130 by targeting its 3′UTR To explore the mechanism by which miR-17-5p induces tumour progression, we used two algorithms that predict mRNA targets: miRNA-PicTar and TargetScan. Based on the frequencies of miR-17-5p sites in their 3′UTRs, >200 mRNAs were predicted to be regulated by miR-17-5p. Gene ontology revealed that these targets included a disproportionately large number of genes encoding proteins with roles in motility-related processes, such as cell adhesion, cytoskeletal remodelling and cell polarity. Guided by this gene ontology analysis, we evaluated eight putative miR-17-5p targets (HBP1, MKK4, P130, PTEN, AIB1, TSG, MAPK9 and STAT3) and two targets (E2F1 and c-Myc) [9] , [13] , [18] that have previously been shown to be involved in tumorigenesis and progression, by investigating the mRNA-level effects of miR-17-5p overexpression and inhibition on these genes in LoVo cells through using qRT–PCR ( Fig. 4a ). Transfecting the LoVo cells with an miR-17-5p mimic significantly decreased the P130 mRNA levels, whereas transfecting the LoVo cells with an miR-17-5p inhibitor significantly increased the P130 mRNA levels. In addition, the data obtained for the two previously validated targets (E2F1 and c-Myc) were consistent with the previously published studies [9] , [13] , [18] . Therefore, we did not select those targets for further analysis in the current study. Similar results were observed in the SW480 cells ( Fig. 4b ). The bioinformatic analysis using the RNA22 program indicated that P130 contains two 3′-UTR elements that are partly complementary to miR-17-5p. 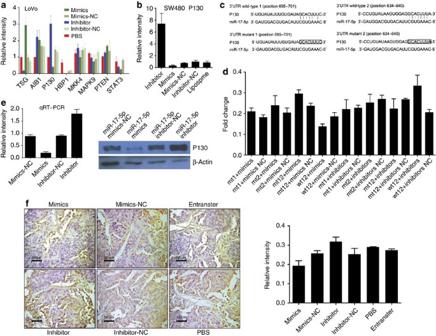Figure 4: miR-17-5p directly targets theP130genein vitroandin vivo. (a) Real-time PCR analysis of the predicted miR-17-5p target genes in the different treatment groups. (b) Real-time PCR analysis for P130 expression levels in the different treatment groups. (c) The putative miR-17-5p-binding site in the P130 3′UTR. (d) The miR-17-5p-binding site in the P130 3′UTR was confirmed in the LoVo cells using a cotransfection luciferase assay for the indicated reporters and the miR-17-5p mimic or for the indicated reporters and the miR-17-5p inhibitor. (e) P130 mRNA and protein levels were determined by qRT–PCR and western blot analyses after injecting the miR-17-5p mimic, mimic control, miR-17-5p inhibitor or inhibitor control into established SW480 CRC xenografts. β-Actin served as the internal control. (f) Immunohistochemisry assay for P130 immunoreactivity in the different treatment groups. These results are representative of at least three independent experiments. All bars represent the mean values±s.d. of three experiments. Figure 4: miR-17-5p directly targets the P130 gene in vitro and in vivo . ( a ) Real-time PCR analysis of the predicted miR-17-5p target genes in the different treatment groups. ( b ) Real-time PCR analysis for P130 expression levels in the different treatment groups. ( c ) The putative miR-17-5p-binding site in the P130 3′UTR. ( d ) The miR-17-5p-binding site in the P130 3′UTR was confirmed in the LoVo cells using a cotransfection luciferase assay for the indicated reporters and the miR-17-5p mimic or for the indicated reporters and the miR-17-5p inhibitor. ( e ) P130 mRNA and protein levels were determined by qRT–PCR and western blot analyses after injecting the miR-17-5p mimic, mimic control, miR-17-5p inhibitor or inhibitor control into established SW480 CRC xenografts. β-Actin served as the internal control. ( f ) Immunohistochemisry assay for P130 immunoreactivity in the different treatment groups. These results are representative of at least three independent experiments. All bars represent the mean values±s.d. of three experiments. Full size image To determine whether P130 is regulated by miR-17-5p through direct binding of its 3′-UTR, we constructed P130 mRNA 3′-UTR fragments (either wild type or mutant) and inserted them immediately downstream of the luciferase reporter gene ( Fig. 4c ). In the luciferase assays, the miR-17-5p mimic was co-transfected into the LoVo cells using different 3′-UTR luciferase constructs. miR-17-5p decreased the relative luciferase activity in the wild-type 3′UTR of P130. Further analysis showed that such regulation was sequence specific, as relative luciferase activities did not decrease as sharply in the UTRs with mutant-binding sites as they did in their wild-type counterparts ( Fig. 4d ). In an in vivo experiment with a tumour xenograft model that used SW480 cells, the qRT–PCR and western blotting analysis found that P130 expression at the mRNA and protein levels decreased in the miR-17-5p mimic-treatment group and increased in the miR-17-5p inhibitor-treatment group relative to the controls ( Fig. 4e ). P130 immunoreactivity was readily detected in the cytoplasm and occasionally in the nucleus. The P130 staining intensity decreased in the miR-17-5p mimic-treatment group and increased in the miR-17-5p inhibitor-treatment group relative to the controls ( Fig. 4f ). In addition, immunodeficient BALB/C mice were subcutaneously injected with LoVo cells to validate the current results, and similar results were obtained using the LoVo cells ( Supplementary Fig. S9 ). Taken together, these results suggest that miR-17-5p downregulates P130 expression in large part by directly targeting its 3′UTR. P130 can block the effects of miR-17-5p on CRC cells To better understand the role of P130 in miR-17-5p-mediated tumour progression, we first examined the expression and function of P130 in CRC. Immunohistochemical staining showed that P130 expression was decreased in most of the CRC tumours ( Supplementary Fig. S10a,b ). Furthermore, the P130 protein levels were inversely correlated with miR-17-5p expression ( Supplementary Fig. S10c ). These findings suggested that the decreased P130 expression might have resulted from increased miR-17-5p expression in the CRC cells. To assess the functional contributions of these miR-17-5p targets to the aggressive phenotypes of the cancer cells, we first examined the role of P130 on cell-cycle progression and tumorigenesis in the SW480 and LoVo cells by knocking down P130 with siRNA. The most effective P130-siRNA target sequence was determined to be siRNA-P130-2 ( Fig. 5a ). Notably, the MTT, TUNEL and transwell assays found that, similar to the effects of miR-17-5p overexpression, P130-siRNA was associated with significantly decreased levels of cell apoptosis, accelerated cell-cycle progression and proliferation and enhanced invasive and migratory abilities in the SW480 and LoVo cells ( Fig. 5c–g ; Fig. 6a–g ). To verify the direct relationship between miR-17-5p and P130, we examined whether P130 inhibition could reverse the effects of miR-17-5p inhibitor transfection in rescue experiments using SW480 and LoVo cells. The results revealed that P130-siRNA can partially reverse the effects of miR-17-5p inhibition on the proliferative, apoptotic, invasive and migratory abilities of SW480 cells ( Fig. 7 ). The above evidence indicates that P130 is indeed a functional target of miR-17-5p. 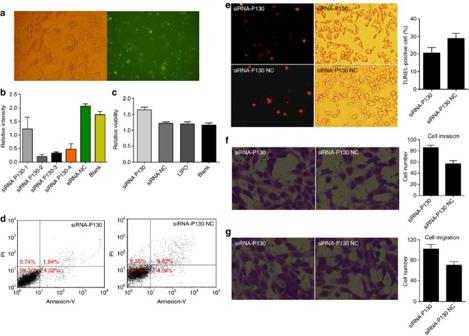Figure 5: P130-siRNA can partly mimic the effects of miR-17-5p on SW480 cells. (a) SW480 cells were transfected with a P130-negative control labelled with a fluorescein amidite molecule. (b) The efficacy of the RNA interference was verified by qRT–PCR analysis of the SW480 cells. (c) P130 downregulation significantly enhanced thein vitrogrowth of the SW480 cells in an MTT assay at 48 h after the transfection. (d) Downregulating P130 significantly inhibited apoptosis in the SW480 cells at 48 h after the transfection. (e) There were significantly fewer TUNEL-positive nuclei in the siRNA-P130-transfected cells than in the control group. (f,g) The transwell assay showed that P130 knockdown markedly increased the invasive and migratory potential of the SW480 cells. These results are representative of at least three independent experiments. All bars represent the mean values±s.d. of three experiments. Figure 5: P130-siRNA can partly mimic the effects of miR-17-5p on SW480 cells. ( a ) SW480 cells were transfected with a P130-negative control labelled with a fluorescein amidite molecule. ( b ) The efficacy of the RNA interference was verified by qRT–PCR analysis of the SW480 cells. ( c ) P130 downregulation significantly enhanced the in vitro growth of the SW480 cells in an MTT assay at 48 h after the transfection. ( d ) Downregulating P130 significantly inhibited apoptosis in the SW480 cells at 48 h after the transfection. ( e ) There were significantly fewer TUNEL-positive nuclei in the siRNA-P130-transfected cells than in the control group. ( f , g ) The transwell assay showed that P130 knockdown markedly increased the invasive and migratory potential of the SW480 cells. These results are representative of at least three independent experiments. All bars represent the mean values±s.d. of three experiments. 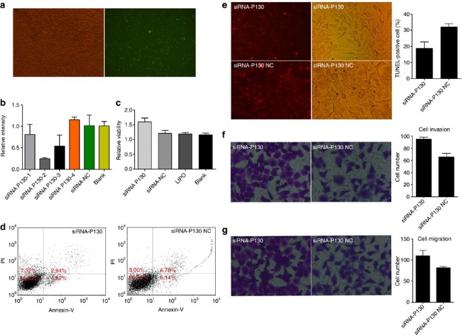Figure 6: P130-siRNA can partially mimic the effects of miR-17-5p on LoVo cells. (a) LoVo cells were transfected with a P130-negative control that had been labelled with a fluorescein amidite molecule. (b) The efficacy of the RNA interference was verified by qRT–PCR analysis of the LoVo cells. (c) MTT assay showed that downregulating P130 significantly enhanced thein vitrogrowth of the LoVo cells at 48 h after transfection. (d) Downregulating P130 significantly inhibited apoptosis in the LoVo cells at 48 h after the transfection. (e) There were significantly fewer TUNEL-positive nuclei in the siRNA-P130-transfected cells than in the control group. (f,g) The transwell assay showed that the P130 knockdown markedly increased the invasive and migratory potential of the LoVo cells. These results are representative of at least three independent experiments. All bars represent the mean values±s.d. of three experiments. Full size image Figure 6: P130-siRNA can partially mimic the effects of miR-17-5p on LoVo cells. ( a ) LoVo cells were transfected with a P130-negative control that had been labelled with a fluorescein amidite molecule. ( b ) The efficacy of the RNA interference was verified by qRT–PCR analysis of the LoVo cells. ( c ) MTT assay showed that downregulating P130 significantly enhanced the in vitro growth of the LoVo cells at 48 h after transfection. ( d ) Downregulating P130 significantly inhibited apoptosis in the LoVo cells at 48 h after the transfection. ( e ) There were significantly fewer TUNEL-positive nuclei in the siRNA-P130-transfected cells than in the control group. ( f , g ) The transwell assay showed that the P130 knockdown markedly increased the invasive and migratory potential of the LoVo cells. These results are representative of at least three independent experiments. All bars represent the mean values±s.d. of three experiments. 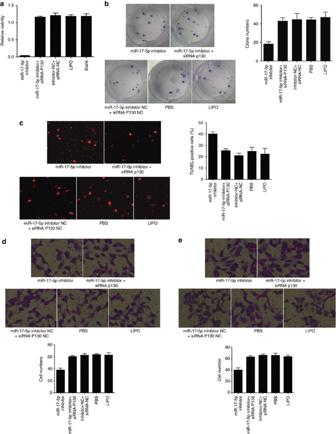Figure 7: P130-siRNA can partially reverse the effects of the miR-17-5p inhibitor on SW480 cells. (a) An MTT assay showed that siRNA-P130 significantly restored the proliferative ability of miR-17-5p inhibitor-transfected SW480 cells. (b) Clonogenic assays showed that siRNA-P130 significantly restored the colony-forming ability of miR-17-5p inhibitor-transfected SW480 cells relative to the negative control. (c) TUNEL assays showed that the siRNA-P130 treatment significantly restored the TUNEL-positive nuclei in the miR-17-5p inhibitor-transfected SW480 cells. (d,e) Transwell assays revealed that the P130-siRNA treatment significantly restored the invasive and migratory capability of miR-17-5p inhibitor-transfected SW480 cells. These results are representative of at least three independent experiments. All bars represent the mean values±s.d. of three experiments. Full size image Figure 7: P130-siRNA can partially reverse the effects of the miR-17-5p inhibitor on SW480 cells. ( a ) An MTT assay showed that siRNA-P130 significantly restored the proliferative ability of miR-17-5p inhibitor-transfected SW480 cells. ( b ) Clonogenic assays showed that siRNA-P130 significantly restored the colony-forming ability of miR-17-5p inhibitor-transfected SW480 cells relative to the negative control. ( c ) TUNEL assays showed that the siRNA-P130 treatment significantly restored the TUNEL-positive nuclei in the miR-17-5p inhibitor-transfected SW480 cells. ( d , e ) Transwell assays revealed that the P130-siRNA treatment significantly restored the invasive and migratory capability of miR-17-5p inhibitor-transfected SW480 cells. These results are representative of at least three independent experiments. All bars represent the mean values±s.d. of three experiments. Full size image miR-17-5p regulates the Wnt/β-catenin signalling pathway Recent research has indicated that aberrant Wnt/β-catenin signalling plays an important role in CRC. The essential event in Wnt signalling is stabilization of β-catenin. Therefore, β-catenin expression levels were investigated in SW480 and LoVo cells by transfection with an miR-17-5p mimic or suppressing P130 with P130-siRNA. The results showed that overexpressing miR-17-5p or suppressing P130 increased β-catenin expression. An in vivo experiment using an SW480-cell tumour xenograft model found that β-catenin expression was higher in the miR-17-5p mimic-treatment group and lower in the miR-17-5p inhibitor-treatment group than in the controls. The effects of significantly inhibiting β-catenin expression levels in CRC cells by using an miR-17-5p inhibitor were assessed ( Fig. 8a ). In addition, immunodeficient BALB/C mice were subcutaneously injected with LoVo cells to validate the current results, and similar results were obtained ( Supplementary Fig. S11 ). These results suggest that miR-17-5p upregulates β-catenin expression in large part by directly downregulating its target gene, P130 ( Fig. 8c ). Together, these data indicate that the ability of miR-17-5p to enhance proliferation, apoptosis, cell-cycle progression, invasion and migration is in large part attributable to its ability to inhibit P130 and subsequently increase β-catenin expression levels. 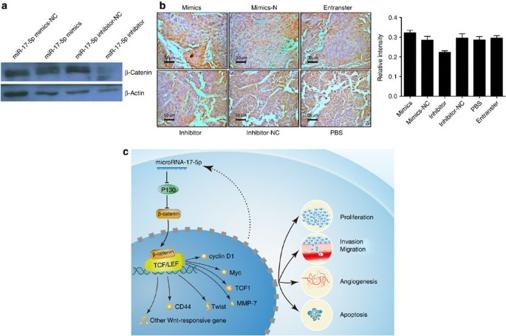Figure 8: miR-17-5p targets the P130-Wnt/β-catenin pathway. (a) β-Catenin protein levels were determined by western blot analysis after injecting an miR-17-5p mimic, a mimic control, an miR-17-5p inhibitor or an inhibitor control into established SW480 CRC cell xenografts. Significant inhibition of β-catenin expression levels by the miR-17-5p inhibitor was found in CRC cells. β-Actin served as an internal control. (b) Significant inhibition of β-catenin expression levels by the miR-17-5p inhibitor was observed in the β-catenin immunoreactivity analysis. The values shown are the average percentages of β-catenin-positive cells counted in five random fields. (c) miR-17-5p enhances CRC cell proliferation, invasiveness and metastasis and inhibits CRC cell apoptosis by directly inhibiting P130 and consequently increasing Wnt/β-catenin expression. These results are representative of at least three independent experiments. All bars represent the mean values±s.d. of three experiments. Figure 8: miR-17-5p targets the P130-Wnt/β-catenin pathway. ( a ) β-Catenin protein levels were determined by western blot analysis after injecting an miR-17-5p mimic, a mimic control, an miR-17-5p inhibitor or an inhibitor control into established SW480 CRC cell xenografts. Significant inhibition of β-catenin expression levels by the miR-17-5p inhibitor was found in CRC cells. β-Actin served as an internal control. ( b ) Significant inhibition of β-catenin expression levels by the miR-17-5p inhibitor was observed in the β-catenin immunoreactivity analysis. The values shown are the average percentages of β-catenin-positive cells counted in five random fields. ( c ) miR-17-5p enhances CRC cell proliferation, invasiveness and metastasis and inhibits CRC cell apoptosis by directly inhibiting P130 and consequently increasing Wnt/β-catenin expression. These results are representative of at least three independent experiments. All bars represent the mean values±s.d. of three experiments. Full size image In the current study, we compared the miRNA profiles of foetal colorectal, CRC and normal colorectal tissues using two screening methods: the μParaflo miRNA microarray and an miRNA cancer array employing the Quantimir system. A total of 39 miRNAs were found to be differentially expressed across the three groups. Most of these miRNAs are involved in biological processes that usually have key roles in both early development and malignant progression. To our knowledge, certain cancer biomarkers with high diagnostic values have embryonic characteristics [19] . These molecules are highly expressed in both foetal and human tumour tissues but are seldom expressed in normal adult tissues. Indeed, it has been widely observed that these genes and proteins are shared between the embryogenesis and tumorigenesis processes [20] . The increased proliferation rate and lack of differentiation in cancer cells resemble the physiological process of embryogenesis [10] . Following this theory, we focused on miRNAs that are more highly expressed in both foetal and CRC tissues than in normal tissues. Only one oncofoetal miRNA, miR-17-5p, was identified. Therefore, miR-17-5p became the focus of this study. miR-17-5p is the main effector of the miR-17-92 cluster component, which has been identified as a member of the solid cancer miRNA signature [21] . In addition to targeting E2F1 and c-Myc [9] , [13] , [18] , miR-17-5p regulates p21, PTEN and BIM expression and functions as a key oncogenic factor [22] , [23] . The present study investigated the mechanism by which miR-17-5p exerts its function and modulates malignant CRC phenotypes in vitro and in vivo . The current data clearly indicated that silencing miR-17-5p expression inhibited CRC cell proliferation, cell migration and invasion and induced in vitro and in vivo cell apoptosis by targeting the P130/β-catenin pathway. miR-17-5p over-expression in CRC cells promoted proliferation, migration and invasion and repressed apoptosis by targeting the P130/β-catenin pathway. These findings suggest that miR-17-5p has an important role in CRC tumorigenesis and progression by suppressing P130 and subsequently activating Wnt/β-catenin. The present data clearly indicated that inhibiting miR-17-5p inhibited in vitro cell proliferation, induced cell apoptosis and inhibited cell migration and invasion in human CRC cells. Moreover, we observed the effects of miR-17-5p inhibition on a tumour xenograft model. It was noteworthy that, consistent with the in vitro outcomes, inhibiting miR-17-5p in vivo was shown to decrease tumour growth, inhibit cell proliferation and induce apoptosis. Consequently, there is a clear indication that miR-17-5p is a promising novel CRC therapeutic target that offers an attractive approach for further investigation. Our findings also support a causal role for altered miR-17-5p expression during tumorigenesis. In the present study, we demonstrated an association between miR-17-5p expression levels and both CRC prognosis and therapeutic outcome. A robust association between high miR-17-5p expression in tumours and poor survival was found in the 240 CRC patients of cohort 1 using qRT–PCR and in the 185 CRC patients of cohort 2 using ISH analysis. The association was independent of other clinical covariates, indicating that miR-17-5p expression may be a useful prognostic biomarker that may help identify patients at higher risk for terminal CRC. However, we demonstrated that high miR-17-5p expression in tumours was associated with a favourable response to adjuvant chemotherapy. This association could help predict the benefits of therapy in individuals whose miR-17-5p expression status is known and help identify patients who are candidates for more aggressive initial therapies. To further explain this phenomenon, we performed an in vitro experiment using two CRC cell lines: LoVo and SW480. We found that the miR-17-5p expression levels were decreased in the cells treated with 5-Fu. In addition, the apoptosis and TUNEL assays confirmed that miR-17-5p suppressed cell apoptosis and G1 arrest but that cell apoptosis and G1 arrest were promoted in the miR-17-5p-transfected CRC cells treated with 5-Fu. These results are consistent with those of a previously published study [24] . However, further research must be performed to unravel the underlying mechanisms. To further study the potential role of miR-17-5p as a biomarker for progression or other aggressive behaviours in CRC, we examined the correlation between miR-17-5p expression and TNM staging and lymph node metastasis. There was a dose–response relationship in the CRC patients: the more advanced tumours expressed higher miR-17-5p levels. miR-17-5p overexpression was more likely to be present in the CRC patients with lymph node metastases. All of these data are consistent with a role for miR-17-5p in colorectal carcinogenesis and progression. In conclusion, miRNA profile screening and molecular, biological and clinical experiments identified miR-17-5p as a potential oncofoetal biomarker for diagnosis, prognosis and therapeutic response in CRC. The current findings suggest that miR-17-5p is a crucial determinant of progression in CRC. Clinical specimens collection Fresh CRC tissues were obtained from eight CRC patients who underwent surgical resections at the Department of Surgery, the Sixth People’s Hospital affiliated to Shanghai Jiao Tong University from 2008 to 2009. Detailed clinical information for the eight fresh samples is shown in Supplementary Table S5 . Eight adenoma colorectal tissues were obtained from the Department of Digestive Endoscopy, and normal colorectal tissue samples were obtained from eight disease-free colorectal donors. Eight foetal colorectal specimens that had been obtained within 4 months were obtained from the Department of Gynaecology and Obstetrics. The eight fresh foetal samples used in the current study were obtained from the colon tissues of embryos up to 4 months after conception. The CRC diagnoses for cohort 1 were confirmed by using qRT–PCR on paraffin-embedded specimens from CRC tissue and the surrounding non-tumour tissues obtained from 240 patients who underwent surgical resections from 2001 to 2007. A summary of the clinical information for these patients in cohort 1 is shown in Supplementary Table S2 . Cohort 2 was investigated using ISH with paraffin-embedded specimens from CRC and the surrounding non-tumour tissues obtained from an independent group of 185 patients who underwent surgical resections from 2003 to 2007. A summary of the clinical information for the patients in cohort 2 is shown in Supplementary Table S2 . Samples from patients with familial adenomatous polyposis or human non-polyposis CRC were excluded from this study. The final follow-up date was 30 April 2010. The project was approved by the institutional review board of the Sixth People’s Hospital (affiliated with Shanghai Jiao Tong University), China. Written informed consent was obtained from all of the patients and tissue sample donors, and anonymity was assured by tracking the patients through their clinical history numbers. RNA isolation and miRNA profiling Total RNA was extracted from tissue samples using the Qiagen Rneasy kit (Qiagen GmbH, Germany) according to the manufacturer’s instructions. The miRNA microarray profiling was performed as previously described. Cancer miRNA array assay miRNA profiling was performed using the cancer miRNA array of the QuantiMir system (System Biosciences, Mountain View, California, USA), which is a real-time PCR-based array containing a panel of 95 cancer-related miRNA assays and the U6 transcript as a normalization signal. The assays were performed as previously described. Quantitative RT–PCR A qRT–PCR for miR-17-5p was performed using SYBRRPremix Ex TaqTM miRNA assays (TakaRa) according to the manufacturer’s instructions and using a 7,500 Real-Time PCR system with small nuclear RNA U6 expression levels as the normalization control. ISH analysis The miRCURY LNA miRNA detection probes for human miR-17-5p, scramble and U6 were purchased from Exiqon. These probes have high affinity and discrimination, enabling specific and sensitive detection of miR-17-5p. ISH was performed using a version of the manufacturer’s protocol for formalin-fixed paraffin-embedded tissue. Cell transfections The LoVo cells were grown in F-12K with 10% foetal bovine serum in a humidified atmosphere containing 5% CO 2 at 37 °C. All of the oligonucleotides (the miR-17-5p mimic, 5′-CAAAGUGCUUACAGUGCAGGUAG-3′, and the miR-17-5p inhibitor, 5′-CUACCUGCACUGUAAGCACUUUG-3′) were obtained from Gene-Pharma (China) and were chemically modified (20-O-Methyl), with confirmed long-term (2 weeks) effects and high gene-knockout efficiency. The LoVo cells were transfected with the oligonucleotides, using Lipofectamine 2000 (Invitrogen, USA) in the indicated concentrations according to the manufacturer’s recommendations. MTT assay The LoVo cells were seeded in triplicate in 96-well plates and transfected with the miR-17-5p mimics, miR-17-5p mimics-NC, miR-17-5p inhibitor or miR-17-5p inhibitor-NC. After incubation at 37 °C for the indicated duration, 20 μl of MTT (2 mg ml −1 , Sigma, St Louis, MO) was added and another 4-h incubation was performed. The formazan MTT precipitate was then dissolved in 200 μl of dimethylsulphoxide, and the absorbance was measured at a wavelength of 490 nm. Clonogenic assay A total of 100 LoVo cells that had been transfected with the miR-17-5p mimic, miR-17-5p mimic-NC, miR-17-5p inhibitor or miR-17-5p inhibitor-NC were seeded in 10-cm dishes. After 2 weeks, the cells were washed with phosphate-buffered saline (PBS) and stained with 0.5% crystal violet in 20% methanol and the number of colonies was counted after 20 min. TUNEL assay The apoptotic cells were identified using an In Situ Cell Death Detection kit (TMR Red, Roche) following the manufacturer’s instructions. Briefly, the SW480 and LoVo cells were placed on cover slips after being transfected with the miR-17-5p mimic, miR-17-5p mimic-NC, miR-17-5p inhibitor, miR-17-5p inhibitor-NC or PBS for 24 h. The cells were then fixed with 4% paraformaldehyde for 1 h, and the sections were washed with PBS, permeabilized with 0.1% Triton X-100 in 0.1% sodium citrate in water for 2 min and washed twice with PBS. A TUNEL reagent was added for 1.5 h in the dark at room temperature. The positive and negative controls were established according to the manufacturer’s instructions. The images were captured on an Olympus microfluorescence microscope. The fluorescence intensity of the TUNEL staining was calculated in four or five sections. Formalin-fixed sections of tumour tissue (5 μM) were deparaffinized in xylene and hydrated in graded ethanol. The apoptotic cells were identified using a Cell Death Detection kit (KeyGen, China) according to the manufacturer’s instructions. Briefly, the sections were incubated with 15 g ml −1 proteinase K for 15 min at room temperature and washed with PBS. The endogenous peroxidase was inactivated by incubating the sections with 3% H 2 O 2 for 5 min at room temperature and then washing with PBS. The sections were immersed in terminal deoxynucleotidyl transferase (TdT) buffer containing deoxynucleotidyl transferase and biotinylated dUTP in TdT buffer, incubated in a humid atmosphere at 37 °C for 90 min, and then washed with PBS. The sections were incubated at room temperature for 30 min with anti-horseradish peroxidase-conjugated antibody, and the signals were visualized with diaminobenzidine; haematoxylin was used as a counter stain. Flow cytometry analysis Apoptosis was assessed by measuring the membrane redistribution of phosphatidylserine with an annexin V-propidium iodide apoptosis detection kit (Sigma, USA). In addition, the propidium iodide-stained LoVo cells were analysed on an EPICS ELITE ESP flow cytometer (Beckman Coulter, USA). Cell migration and invasion assays Cell migration and invasion were detected using transwell chambers (8 μm, Corning Costar Co., Cambridge, MA). 5-Fu treatment assay At 24 h after transfection with the miR-17-5p mimic, miR-17-5p mimic-NC, miR-17-5p inhibitor, miR-17-5p inhibitor-NC and PBS, all of the cell lines were plated in triplicate in 96-well plates at 5 × 10 3 cells per well. After 24 h, an additional 100 μl of medium containing 5-Fu was added, and the cells were cultured for an additional 72 h. The concentration of 5-Fu varied between 0.5 × 10 −6 and 30 × 10 −6 mol l −1 . Luciferase target assay A total of 5.0 × 10 4 cells in 24-well plates were co-transfected with 0.6 μg of the indicated pRLTK renilla luciferase construct, 60 ng of pGL3 firefly luciferase normalization control, 200 nM of the miR-17-5p mimic or inhibitor or the corresponding control. The lysates were collected 48 h after transfection, and both the renilla and firefly luciferase activities were measured with a Dual-Luciferase Reporter System (Promega). Immunohistochemistry and histological examination For the immunohistochemistry, the sections were deparaffinized and rehydrated, and the antigens were retrieved by boiling the samples in a citrate buffer for 15 min at 92–98 °C and trypsinizing with 0.125% trypsin for 15 min at 37 °C. The sections were immersed in 3% hydrogen peroxide and distilled water for 30 min to block the endogenous peroxidase activity. Non-specific staining was eliminated by a 20-min incubation with normal sheep serum (DAKO Corp. USA). The sections were incubated with rabbit anti-human PCNA antibody (1:125 dilution; Abcam, Cambridge, UK) at 37 °C for 2 h and then incubated with goat anti-rabbit secondary antibodies (IgG/HRP) for 15 min at 37 °C using Non-Bio Two-Step Histostain-Plus kits, DAB staining (Zhongshan Goldenbridge Biotechnology, Corp. Beijing, China). The nuclei were counterstained with haematoxylin. The remaining procedures were performed in accordance with the manufacturer’s instructions. The immunohistochemically stained sections were observed under light microscopy. Statistical analyses The statistical analyses were performed using GraphPad Prism (GraphPad Prism Software, Version 5.01, GraphPad, San Diego, CA) and SPSS for Windows version 15.0.0 (SPSS, Inc., USA) software packages. Comparisons between the two groups were performed using the Student’s t -test, Dunnett- t -test, or Mann–Whitney test, where appropriate, and comparisons among multiple groups were performed using a one-way analysis of variance model. The survival curves were generated according to the Kaplan–Meier method, and the statistical analyses were performed using the log-rank test. The multivariate analyses used Cox proportional hazards models. Significance was defined as P <0.05. The experimental methods are described in detail in the Supplementary Information. How to cite this article: Ma, A. et al. Elevated oncofoetal miR-17-5p expression regulates colorectal cancer progression by repressing its target gene P130. Nat. Commun. 3:1291 doi: 10.1038/ncomms2276 (2012).